On the problems and promises of savanna fire regime change 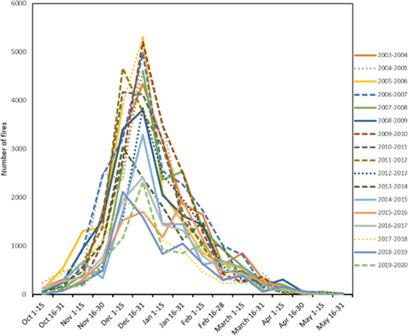Fig. 1: Number of active fires for an area of mesic savanna in West Africa covering portions of Mali, Guinea, Burkina Faso, and Ivory Coast with 750–1000 mm precipitation detected by MODIS over 15 years9. Note the high degree of regularity with a large number of fires lit early (prior to the government’s early fire cut-off of January 1). The recently documented decrease in fire is also apparent24. 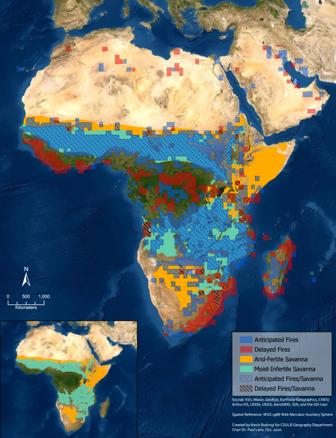Fig. 2: Map of early (anticipated) and late (delayed) fire seasons for Africa modified from Le page et al.7over White’s savanna vegetation map25. Using threshold at ±30 days of difference between the values per grid cell for the middle of the fire season and middle of the CBI season, less than 6% of African savannas burn late. (Sources: Source: Esri, Maxar, GeoEye, Earthstar Geographics, CNES/ Airbus DS, USDA, USGS, AeroGRID, IGN, and the GIS User Community. Created by Kevin Bodrogi). GHG emissions from fires, such as methane, are determined by multiple factors, many of which change by season, but the proposed model only considers changes in the area burned. Critically, the model does not take into account the seasonal changes in EFs. In Africa, for example, EFCH 4 increases by 50–400% when fires are earlier due to higher fuel moisture content [2] , [3] , [4] , [5] . As such, efforts to reduce emissions by burning earlier are misguided because the reduction in the burned area would be offset by the increase in EF resulting in higher methane emissions [4] . Indeed, authors of the Australian research, on which the model is based, have stated as much [6] . In Africa, EDS burning is already widely practiced—the number and extent of fires typically peak prior to the middle of the dry season in the major savanna belts (see below) [7] , [8] . The temporal pattern of burning is very regular, indicating a systematic regime of EDS burning as shown in Fig. 1 for a sub-set of the mesic savanna belt in West Africa. This pattern reflects an intensive effort by thousands of people to set fires early and systematically [7] , [8] , [9] . The regular annual pattern is a function of people selecting and burning specific patches of vegetation that are just dry enough to burn [10] , [11] . These regimes of burning create patch-mosaics of previously burned, newly burned, and unburned vegetation—a process which reflects how the well-timed fires burn only grasses that have sufficiently cured, leaving the adjacent uncured grasses unburned [8] , [10] . As such, we question that additional vegetation could be burned early and wonder who would do the burning, and what would be the emissions impact of burning more uncured grasses? Importantly, increasing EDS burned area may not be possible due to both ecological (e.g., prevalence of too moist perennial grasses) and socio-economic factors, including constraints posed by agriculture. Increasing the amount of area burned early would require more fires being set during the harvest season and would undoubtedly result in crop damage [12] . Fig. 1: Number of active fires for an area of mesic savanna in West Africa covering portions of Mali, Guinea, Burkina Faso, and Ivory Coast with 750–1000 mm precipitation detected by MODIS over 15 years [9] . Note the high degree of regularity with a large number of fires lit early (prior to the government’s early fire cut-off of January 1). The recently documented decrease in fire is also apparent [24] . Full size image At the core of the proposed model is the application of an early/late fire dichotomy, which itself derives from a series of colonial-era experiments conducted in Africa and later repeated globally. These works examined the impacts of fires set near the beginning and end of the fire season, not the middle, which is when most fires occur [13] . Emissions from fires are a function of a suite of variables that are associated with fuel conditions and weather, which determine the key fire characteristics. These vary by season (as well as spatially) and by fire type. Wind, to give just one example, is critical and peaks in the middle season in parts of Africa. Research also finds that fire type (head or back) has a significant impact on fire intensity, combustion efficiency, and methane EF, yet no mention of fire type appears in the policy [14] . Critically, the authors offer no justification for their crude method of using months of least rainfall to distinguish early from late burning. There are far better alternatives such as vegetation dryness indexes [15] or the Chandler Burning Index (CBI) both of which have been measured remotely and which provide a good indication of fuel moisture level at a scale reasonable for determining potential fire conditions. Indeed, Le Page et al. analyzed the timing of fire regimes globally compared to peak biomass dryness using CBI. They found that most African savannas burn at least 30 days prior to peak dryness (Fig. 2 ) [7] . This figure is in stark contrast with that used by Lipsett-Moore et al., which shows many savanna countries with predominantly LDS fire regimes. It is also noteworthy that Le Page used a grid-cell basis for their analysis that more accurately estimates the conditions of the fuels, compared with the crude country-level estimates based on rainfall used by Lipsett-Moore et al. Fig. 2: Map of early (anticipated) and late (delayed) fire seasons for Africa modified from Le page et al. [7] over White’s savanna vegetation map [25] . Using threshold at ±30 days of difference between the values per grid cell for the middle of the fire season and middle of the CBI season, less than 6% of African savannas burn late. (Sources: Source: Esri, Maxar, GeoEye, Earthstar Geographics, CNES/ Airbus DS, USDA, USGS, AeroGRID, IGN, and the GIS User Community. Created by Kevin Bodrogi). Full size image It is well-documented that mapping of burned areas produced by a regime of patchy fires contains high levels of uncertainty; what is less well-known is that most patch-mosaic burning begins early. Although algorithms to estimate burned areas have improved, the commonly used ones tend to underestimate smaller fires resulting in significant underestimates of burned area and emissions from fires in Africa [16] . Critically, the fires missed are most often early, patchy ones [17] posing two problems for the model. First, existing maps likely underestimate the amount of early burning making the use of a simple EDS/LDS ratio biased. And second, it would be difficult to monitor any shift in burning resulting from a policy change. The proposed policy for a regime of early burning is hardly new but has been practiced in Africa before. French and British colonial foresters also considered early fire preferable to late and when they did, colonial powers promoted a burning regime that was already widely practiced by the indigenous population. Our research documented how French foresters, realizing the impossibility of fire suppression, shifted their policy to promote early fires—a practice developed and used first by Africans [18] . Although well-intended, the model to reduce GHG emissions by selecting countries based on their presumed high LDS fire is flawed and unlikely to succeed. Indeed, if the numbers used by the IPCC are correct, a shift to earlier fires would cause an increase in methane emissions due to increased burning of uncured fuels. Rather than rework the proposed model, we suggest a better approach begins with the wealth of existing studies that seek solutions combining local practice with forestry department objectives [19] , [20] . In addition, it is critical to remember, that the existing burning regimes of Africans serve a plethora of purposes including reducing fire hazards and supporting biodiversity [10] . The types of fires which preserve human livelihoods and biodiversity are not always aligned with the goal of reducing GHG concentrations [8] . As such, changes in burning may result in unforeseen negative consequences [21] . Finally, recent research from Australia, where the proposed model originates, cautions against overly simple solutions to the fire emissions problem [22] . We agree there is a need to modify fire regimes to reduce LDS fires in some places. Indeed, we often find this to be a goal of local populations. In cases we have studied, changing fire is not a matter of simply increasing early fire, but a complex management goal requiring strategies to maximize the good aspects of fire while minimizing the bad ones in accordance with local desires. A better approach would be to begin by studying how African people use strategic burning to render the landscape useful; only then can we begin to work with people to understand their needs and jointly develop methods to prevent unwanted fires. This will require collaborative efforts, community organizing, and smart technologies such as drones for mapping and smartphones for improving communication. We end by noting the irony of the proposed solution of an EDS fire policy for the Australian context. This is, in effect, an effort to reintroduce the fire regime that was lost when the Aboriginal burning practices were suppressed and people were removed from the landscape [23] . In Africa, where the practice of EDS fires has largely persisted—in spite of suppression efforts—we suggest compensating the thousands of people for the ecosystem services they provide by setting fires early.